Spatial organization of frequency preference and selectivity in the human inferior colliculus To date, the functional organization of human auditory subcortical structures can only be inferred from animal models. Here we use high-resolution functional magnetic resonance imaging at ultra-high magnetic fields (7T) to map the organization of spectral responses in the human inferior colliculus, a subcortical structure fundamental for sound processing. We reveal a tonotopic map with a spatial gradient of preferred frequencies approximately oriented from dorsolateral (low frequencies) to ventromedial (high frequencies) locations. Furthermore, we observe a spatial organization of spectral selectivity (tuning) of functional magnetic resonance imaging responses in the human inferior colliculus. Along isofrequency contours, functional magnetic resonance imaging tuning is narrowest in central locations and broadest in the surrounding regions. Finally, by comparing subcortical and cortical auditory areas we show that functional magnetic resonance imaging tuning is narrower in human inferior colliculus than on the cortical surface. Our findings pave the way to noninvasive investigations of sound processing in human subcortical nuclei and for studying the interplay between subcortical and cortical neuronal populations. The inferior colliculus (IC)—centrally located in the auditory pathway—is an obligatory relay station for all information ascending from brainstem nuclei to thalamus and cortex [1] . The IC is pivotal for a vast number of auditory tasks [2] , [3] , [4] , [5] and thus, understanding its functional organization is key in advancing knowledge on how sound perception emerges in the human brain. The functional organization of the IC has been investigated in a variety of non-human species (for example rats, cats, squirrel monkey) using invasive electrophysiological recordings [1] , [6] , [7] , [8] and, more recently, non-invasively using functional magnetic resonance imaging (fMRI) [9] , [10] . Various studies showed that the IC is tonotopically organized [1] . In the rat and in the cat, the orientation of the main tonotopic gradient (low-to-high frequency preference) is orthogonal to the fibrodendritic laminae in the central nucleus of the IC [6] , [11] and runs in the dorsolateral to ventromedial direction [7] . On the basis of these results in animals and on the observation of tonotopic maps in the human cortex [12] , [13] , [14] , [15] , [16] , [17] , [18] , the human IC (hIC) is assumed to be tonotopically organized as well. However, there is no experimental evidence for the existence and spatial layout of a tonotopic map of hIC. Furthermore, in humans, it is unknown whether selectivity of spectral tuning (that is tuning width) is homogeneous or location-dependent throughout the hIC, a question so far addressed only by studies in the cat IC [8] . Finally, although electrophysiological recordings revealed fine frequency tuning in the human and animal auditory cortex [19] , no information is available to compare tuning width between the human midbrain and cortex in response to the same stimuli. In the present study, we examined the spatial organization of spectral responses in hIC using fMRI at 7T. Our analysis of fMRI responses to simple tones and natural sounds revealed the detailed layout of the tonotopic organization within hIC. Furthermore, the estimation of voxels’ spectral response profiles (SRP) with mathematical modelling of the fMRI responses to the natural sounds (that is fMRI encoding [20] , [21] , [22] , [23] ) enabled us to map the spectral selectivity of different locations in the hIC (fMRI tuning) and compare it with that of primary and non-primary auditory cortical areas. fMRI best-frequency maps in the hIC In three distinct experiments, we acquired high-resolution (1.5 mm isotropic) fMRI data (five subjects participated in both Experiment 1 and 2 and four different subjects participated in Experiment 3) covering the brain transversally from the inferior portion of the temporal pole to the superior portion of the superior temporal gyrus (STG) bilaterally ( Supplementary Fig. S1 ). In Experiment 1 and 3, auditory stimuli were 800 ms long amplitude-modulated (8 Hz) tones grouped in blocks around three or eight centre frequencies (0.5; 1.5; 2.5 KHz, Experiment 1; 0.18; 0.30; 0.51; 0.86; 1.46; 2.48; 4.19; 7.09 KHz, Experiment 3). In Experiment 2, a large collection of natural sounds was presented randomly (for example speech segments, musical instruments, animal cries; all 1 s duration). To ensure clear perception of the stimuli, all sounds were presented (at~60 dB sound pressure level) in silent gaps between the acquisitions of subsequent brain volumes see Supplementary Information for details). We computed statistical activation maps for each tone condition (Experiment 1 and 3) or each sound (Experiment 2) ( Supplementary Information ). In all subjects, we observed reliable bilateral activation of the IC [10] , [24] , [25] . The medial geniculate nucleus of the thalamus was less consistently activated (in two of the subjects bilaterally, and two subjects only unilaterally; see Supplementary Fig. S2 for an example), and therefore was excluded from further analysis. Furthermore, we observed consistent activation in the auditory cortex, including the Heschl’s region (approximately corresponding to the primary auditory core) [13] , and surrounding regions in the planum temporale and STG (posterior and anterior) ( Supplementary Fig. S3 ; group activation maps). We derived tonotopic (best-frequency) maps ( Figs 1 and 2 ) by colour coding a voxel according to the tone eliciting the strongest fMRI response (Experiment 1 and Experiment 3) or to the peak-frequency of its haemodynamic SRP calculated with natural sounds (Experiment 2; see Supplementary Information for details). Although not identical, tonotopic maps obtained from tones (Experiment 1) and natural sounds (Experiment 2) were similar as highlighted by a spatial correlation analysis at the group level ( r =0.22, 3,602 voxels; P <0.001, permutation testing) and at single-subject level in four of five subjects ( P <0.05, 3,602 voxels, permutation testing). In both tonotopic maps, the spatial distribution of best-frequency progressed approximately from dorsolateral locations (low frequencies, red colour) to ventromedial locations (high frequencies, blue colour). We verified this observation by quantitatively assessing the direction of the main frequency gradient in the maps (Methods and Supplementary Information ). Specifically, we computed the direction of increasing best frequency with respect to a transversal (that is horizontal) vector pointing in the anterior to posterior direction in sagittal slices. This analysis was performed both at individual subject level (grey arrows in Fig. 3 ) and in the group maps (coloured arrows in Fig. 3 ). The main frequency gradient (group maps) was oriented at an angle of 260° (left hemisphere) and 262° (right hemisphere) with respect to the horizontal axis in Experiment 1 (variability of ±10° across sagittal slices), at an angle of 252° (left hemisphere) and 261° (right hemisphere) in Experiment 2 (with a variability of±15° across sagittal slices) and at an angle of 262° (left hemisphere) and 265° (right hemisphere) in Experiment 3 (with a variability of ±10° across sagittal slices). 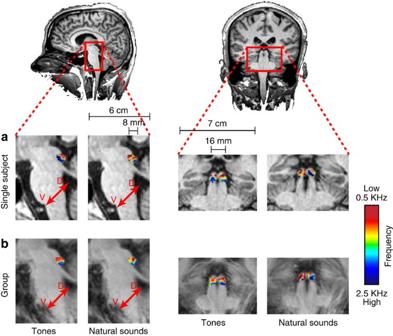Figure 1: Tonotopic maps in the hIC based on Experiments 1 and 2. Maps of frequency preference (tonotopic maps) in the IC for a representative subject (a) and in the group (b) obtained from single tones (three main frequencies, Experiment 1) and natural sounds (Experiment 2). Sagittal (left panel) and coronal (right panel) views of the maps are superimposed on high-resolution anatomical images of the subject (a) and to the anatomical images obtained from the average of all subjects (b). The red arrow in the sagittal sections indicates the dorsal (D) to ventral (V) direction in the human IC. Figure 1: Tonotopic maps in the hIC based on Experiments 1 and 2. Maps of frequency preference (tonotopic maps) in the IC for a representative subject ( a ) and in the group ( b ) obtained from single tones (three main frequencies, Experiment 1) and natural sounds (Experiment 2). Sagittal (left panel) and coronal (right panel) views of the maps are superimposed on high-resolution anatomical images of the subject ( a ) and to the anatomical images obtained from the average of all subjects ( b ). The red arrow in the sagittal sections indicates the dorsal (D) to ventral (V) direction in the human IC. 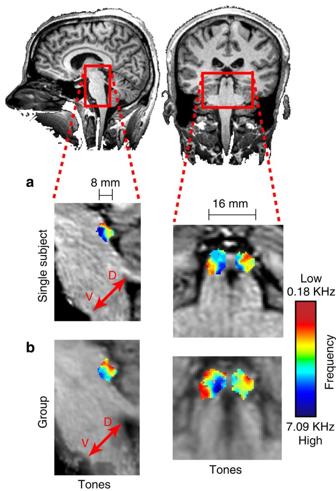Figure 2: Tonotopic maps in the hIC based on Experiment 2. Maps of frequency preference (tonotopic maps) in the IC for a representative subject (a) and in the group (b) obtained from single tones (eight centre frequencies, Experiment 3). Sagittal and coronal views of the maps are superimposed on high-resolution anatomical images of the subject (a) and to the anatomical images obtained from the average of all subjects (b). The red arrow in the sagittal sections indicates the dorsal (D) to ventral (V) direction in the human IC. Full size image Figure 2: Tonotopic maps in the hIC based on Experiment 2. Maps of frequency preference (tonotopic maps) in the IC for a representative subject ( a ) and in the group ( b ) obtained from single tones (eight centre frequencies, Experiment 3). Sagittal and coronal views of the maps are superimposed on high-resolution anatomical images of the subject ( a ) and to the anatomical images obtained from the average of all subjects ( b ). The red arrow in the sagittal sections indicates the dorsal (D) to ventral (V) direction in the human IC. 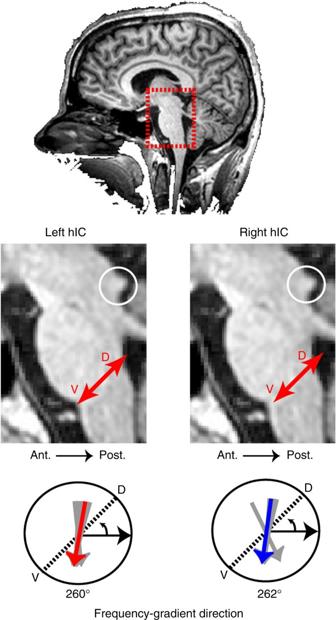Figure 3: Frequency gradient in the hIC. Direction of the frequency gradient in the left and right hIC as obtained from the response to simple tones (Experiment 1). Angles are referred to a vector pointing in the anterior-to-posterior directions as indicated in the figure. Grey arrows indicate single-subject results, and coloured arrows indicated results obtained from the group tonotopic maps. The dorsal (D) to ventral (V) direction in the human IC is indicated by a black dotted line. Full size image Figure 3: Frequency gradient in the hIC. Direction of the frequency gradient in the left and right hIC as obtained from the response to simple tones (Experiment 1). Angles are referred to a vector pointing in the anterior-to-posterior directions as indicated in the figure. Grey arrows indicate single-subject results, and coloured arrows indicated results obtained from the group tonotopic maps. The dorsal (D) to ventral (V) direction in the human IC is indicated by a black dotted line. Full size image fMRI-based frequency tuning in the hIC and cortex From the SRPs estimated in Experiment 2 (natural sounds) we defined the spectral tuning width of fMRI responses as the ratio TW between its best frequency (BF in Hz, the peak of the SRP) and the width of a Gaussian function (full-width at half-maximum (FWHM) in Hz) centred around BF (see Supplementary Information ). Thus, high TW values indicate narrow tuning while low TW values indicate broad tuning. In accordance with previous studies in animals [26] , [27] , we observed a positive correlation between BF and TW. This relationship was removed before interpreting the spatial distribution of tuning width throughout hIC (see Supplementary Information ). The group maps of tuning width are reported in Fig. 4b together with the tonotopic maps ( Fig. 4a ). We observed narrower tuning in central portions of the IC (blue violet in Fig. 4b ) and broadly tuned voxels (yellow orange in Fig. 4b ) on its outer shell. This spatial distribution of fMRI tuning within the hIC was further examined by sampling the tuning width along the isofrequency contour of the middle frequency (1.5 kHz) region in the tonotopic maps obtained from Experiment 1 (group and single-subject map, see Fig. 4c and Supplementary Fig. S4c , respectively). To minimize the variation in length of the isofrequency contours, we selected slices in the centre of the IC and interpolated all isocontours to the average contour length (~8 mm). 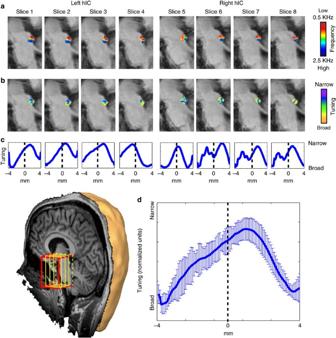Figure 4: Tuning width maps in the hIC. Eight equally spaced sagittal slices (four in the left IC and four in the right IC) of the group tonotopic map (red-yellow-green-blue scale), as obtained in Experiment 1 (‘tones’) superimposed to group-averaged anatomical images (a). Group tuning width map (purple-blue-green-yellow scale), as obtained in Experiment 2 (‘natural sounds’) (b). The map is superimposed to group-averaged anatomical images for the same eight equally spaced sagittal slices presented ina. Spectral tuning sampled along the 1.5 kHz isofrequency line for the same eight equally spaced slices presented ina,b(dashed line marks the centre of the isofrequency line) (c). Averaged distribution (mean and s.d. across slices) of spectral tuning along the 1.5 kHz isofrequency line (d). The dashed line marks the center of the isofrequency line. Figure 4d represents the mean tuning width variation along the isofrequency contour across all slices. Both in single sagittal slices and in mean across the hIC, tuning width was narrower at the centre of the isofrequency contour (high values of TW), and broadened at its outer edges (low values of TW). Results of single-subject analysis revealed the same pattern ( Supplementary Fig. S4 ). This spatial distribution cannot be explained by variations in overall activation levels of IC voxels ( Supplementary Information and Discussion ). Figure 4: Tuning width maps in the hIC. Eight equally spaced sagittal slices (four in the left IC and four in the right IC) of the group tonotopic map (red-yellow-green-blue scale), as obtained in Experiment 1 (‘tones’) superimposed to group-averaged anatomical images ( a ). Group tuning width map (purple-blue-green-yellow scale), as obtained in Experiment 2 (‘natural sounds’) ( b ). The map is superimposed to group-averaged anatomical images for the same eight equally spaced sagittal slices presented in a . Spectral tuning sampled along the 1.5 kHz isofrequency line for the same eight equally spaced slices presented in a , b (dashed line marks the centre of the isofrequency line) ( c ). Averaged distribution (mean and s.d. across slices) of spectral tuning along the 1.5 kHz isofrequency line ( d ). The dashed line marks the center of the isofrequency line. Full size image Cortical tonotopic maps showed a large low-frequency region oriented along the posterior part of HG and bordered anteriorly and posteriorly (on FTS and HS/anterior planum temporale, respectively) by regions preferring higher frequencies ( Supplementary Fig. S5 ; region outlined by white circle in second row). Beyond these main frequency clusters centred on Heschl’s region, we observed additional low and high frequency clusters on PP and STG/STS. In the tuning width maps we observed a region of narrow tuning ( Supplementary Fig. S5 , purple/blue colours in the bottom row) along HG in each hemisphere, surrounded by regions of broader tuning (in yellow/orange). We defined three distinct cortical regions on the superior temporal plane based on the combination of tonotopy (Experiments 1 and 2) and tuning width (Experiment 2 only) maps. Specifically, we defined hA1 and hR as the tonotopically organized and narrowly tuned region situated along Heschl’s gyrus [13] , [28] , and the lateral belt as the more broadly tuned region at the posterior adjacency of hA1 and hR [29] , [30] , [31] ( Supplementary Fig. S5 ). Next, both for hIC and for these three cortical areas, we compared at single-subject level the proportion of narrowly and broadly tuned voxels. To this end, we calculated subject-specific histograms of voxels' TWs in proportional terms of the total number of voxels in each region ( Fig. 5 ). At the single-subject level, we observed a wide distribution of TW values; however, a larger proportion of voxels with narrower tuning was present in the IC (grey curves in Fig. 5 ) compared with all other cortical areas. Although in most subjects the tuning width in cortical regions was limited to 0.6 octaves (TW=2.5) or broader, in the IC several voxels were more narrowly tuned (up to 0.45 octaves; TW=3.23). Finally, we tested whether fMRI tuning was significantly different across regions. First, we defined four intervals equally spaced between the minimum and maximum observed tuning widths. Per interval, we tested the differences in the proportion of voxels across the four regions ( Fig. 6 , Wilcoxon rank sum tests). We observed significant differences between lateral belt and hIC in the narrowest and broadest tuning width bin. The lateral belt contained more broadly tuned voxels than hIC and hR ( P <0.05 ; n =5; Wilcoxon rank sum test), whereas hIC contained more narrowly tuned voxels than lateral belt and hR ( P <0.05 ; n =5; Wilcoxon rank sum test). When testing for differences in mean tuning width between areas across subjects, (Wilcoxon rank sum test), we observed narrower fMRI tuning in the hIC compared with lateral belt areas bilaterally ( P <0.05 ; n =5; Wilcoxon rank sum test), and narrower fMRI tuning in right hIC than in right hA1 ( P <0.05 ; n =5; Wilcoxon rank sum test). 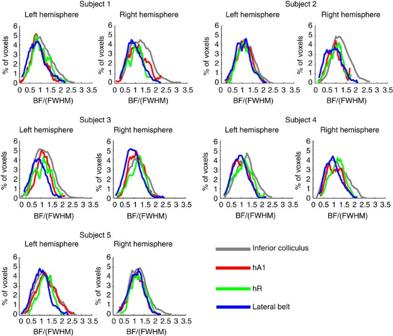Figure 5: Tuning-width distribution in the hIC and cortex. Histograms of voxels’ tuning width (BF in Hz/FWHM in Hz) for each region (IC—grey, hA1—red, hR—green, lateral belt—blue) and hemisphere. Note that a larger proportion of narrowly tuned voxels are present in hIC (grey curves; high values), whereas lateral belt regions contain a larger proportion of broadly tuned voxels (blue curves; low values). Figure 5: Tuning-width distribution in the hIC and cortex. Histograms of voxels’ tuning width (BF in Hz/FWHM in Hz) for each region (IC—grey, hA1—red, hR—green, lateral belt—blue) and hemisphere. Note that a larger proportion of narrowly tuned voxels are present in hIC (grey curves; high values), whereas lateral belt regions contain a larger proportion of broadly tuned voxels (blue curves; low values). 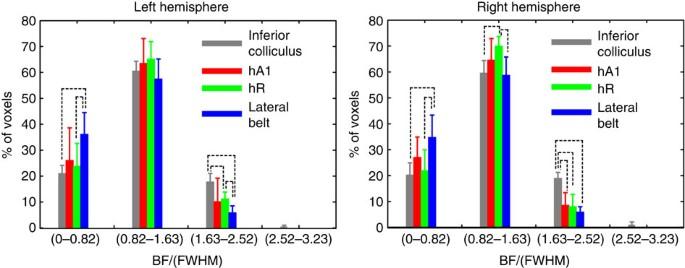Figure 6: Comparison of tuning width distributions of different auditory stages. The percentage of voxels with spectral tuning (BF/FWHM) within four different windows ([0–0.82], [0.82–1.63], [1.63–2.52], [2.52–3.23]) is reported for four different areas (IC—grey, hA1—red, hR—green, lateral belt—blue) in both left (left column) and right (right column) hemispheres. Error bars represent s.d. across subjects. Dashed lines mark significant differences (Wilcoxon rank sum test;P=0.05;n=5). Full size image Figure 6: Comparison of tuning width distributions of different auditory stages. The percentage of voxels with spectral tuning (BF/FWHM) within four different windows ([0–0.82], [0.82–1.63], [1.63–2.52], [2.52–3.23]) is reported for four different areas (IC—grey, hA1—red, hR—green, lateral belt—blue) in both left (left column) and right (right column) hemispheres. Error bars represent s.d. across subjects. Dashed lines mark significant differences (Wilcoxon rank sum test; P =0.05; n =5). Full size image In this study, we used high-resolution fMRI to map the spatial organization of spectral responses in the hIC based on responses to simple tones (Experiment 1 and 3) and natural sounds (Experiment 2). Across subjects and experiments, we consistently observed a low-to-high frequency gradient in hIC, approximately oriented along a dorsolateral to ventromedial direction. Furthermore, spectral selectivity (fMRI tuning) based on responses to natural sounds was organized in a narrow-to-broad tuning pattern when progressing from central to peripheral locations. Finally, we showed that fMRI tuning in hIC was narrower than in primary (right hemisphere) and non-primary auditory (bilaterally) cortical areas. The presence of a tonotopic map in the hIC is consistent with early reports in animals (for example cat and monkey) obtained using invasive electrophysiological recording [7] , [32] and, more recently, with fMRI in the monkey [10] . On the contrary, a recent study in the rhesus monkey IC has questioned the existence of a full tonotopic gradient by showing a small tonotopic region (centre of the IC) surrounded by a large field with a low frequency bias [33] . Our results in humans do not support these findings but are consistent with earlier reports showing a full tonotopic gradient in the IC. The IC frequency gradient observed in non-human species was oriented in a dorsolateral to ventromedial direction [5] , [7] , [8] , [9] , [10] , [32] . In hIC, the dorsal-to-ventral direction runs orthogonal to the direction of the brain stem, at an orientation of 225° relative to the anterior-posterior horizontal axis (that is red arrow in Figs 1 and 2 , and black dotted line in Fig. 3 ). Our analysis revealed a tonotopic gradient oriented at ~260° with respect to the anterior-to-posterior direction, which represents a deviation of 35° with respect to the dorsal-to-ventral direction. It is challenging to say whether this difference reflects an anatomical shift of the colliculus with respect to the brain stem across species or simply results from the inaccurate alignment of previous results with the present maps. The comparison of imaging data across species [10] , [34] , with careful realignment to the same reference system, may enable a more precise comparison. Furthermore, three-dimensional representations of the tonotopic gradient from electrophysiology studies in animals have shown a gradual tilt of the isofrequency laminae in the rostral and lateral directions [7] , [35] . Despite the relatively high spatial resolution of our measurements, we could not detect such a tilt in the orientation of the isofrequency contours within hIC. Instead, our gradient analysis of best-frequency maps was limited to the main frequency gradient (that is averaged across all pixels in sagittal slices of the hIC). Voxels whose best frequency does not follow this principal gradient direction are visible in selected slices, particularly in the tonotopic maps obtained with natural sounds ( Fig. 1 ). We expect that these variations may reflect an irregular spatial distribution of the frequency gradient. Alternatively, they could result from the inaccurate estimation of the voxels’ SRPs. Beyond maps of tonotopy, we revealed a spatial organization of tuning width of haemodynamic responses in hIC. That is, narrow tuning in the centre of the hIC, and broad tuning at its extremes. Given the complexity of the fMRI signal, both vascular and neuronal factors may contribute to this observation. The distribution of fMRI tuning width values did not correlate well with the overall fMRI signal strength, which suggests that the observed radial organization is not likely to result from macroscopic vasculature differences. Nevertheless, this lack of correlation does not exclude the possibility that more subtle vasculature differences within the hIC (for example between its central and lateral portions) may underlie the observed tuning width patterns. Furthermore, it should be considered that we cannot distinguish between the three nuclei comprising the IC. Consequently, the broadly tuned IC regions could also reflect the dorsal or external portion of the IC. Keeping these intrinsic caveats in mind, it is nevertheless noteworthy that the interpretation of our fMRI tuning width maps in terms of neuronal population responses is compatible with reports of spectral tuning width in the cat IC, where tuning width was found to be most narrow on the medial third of frequency band laminae [8] . Future studies may shed light on possible confounds, for example by discriminating hIC subdivisions based on their anatomical connectivity and/or functional properties, which may be assessed noninvasively. In most electrophysiology studies, recordings of neuronal responses are limited to single cortical or midbrain regions and consequently comparing the width of frequency tuning across multiple stages of the auditory pathway remains challenging [36] . The large brain coverage achievable with fMRI allowed us to obtain, within each single subject, tonotopic and tuning width measures in both the hIC and cortex. Over the last decades, cortical tonotopic maps have been reliably extracted using fMRI [13] , [14] , [15] , [16] , [17] , [18] , [37] , [38] , [39] . Tonotopic patterns estimated in these various studies displayed great stability around Heschl’s region, and this pattern is replicated in our group tonotopy maps. In spite of substantial consistency across maps of tonotopy across experiments, their interpretation—and the exact orientation of the primary and other tonotopic gradients with respect to the HG anatomy—is still debated [13] , [15] , [16] , [18] . Several imaging studies suggested that the primary tonotopic gradient is oriented in posteromedial to anterolateral direction along HG [13] , [38] , [39] . Conversely, recent studies argued that the main gradient runs in anterior-to-posterior direction [15] , [18] , [37] , possibly with a curvature between the two principal frequency gradients [16] . Here, we combined maps of tonotopy and tuning width to identify core and lateral belt regions. In the monkey auditory cortex, narrowly tuned primary areas are surrounded by a belt of more broadly tuned non-primary areas [30] , [40] , [41] , [42] , [43] . We interpreted the narrow region as reflecting the core [31] , containing two frequency gradients that may reflect the human homologues of monkey A1 and R [28] , [29] . Comparing, within each single subject, the tuning width of the hIC and auditory cortical regions we observed that the IC had a significantly larger proportion of voxels narrowly tuned compared with the cortex, with the lateral belt exhibiting the largest proportion of broadly tuned voxels. Voxels’ tuning widths as estimated here extended over a wide distribution of values but were limited—at their lower boundary—to values broader than ~1/2 (0.45) of an octave. These results are in apparent contradiction with recent human and monkey electrophysiology data [19] , [36] , which showed cortical spectral tuning width as narrow as 1/12 octave. However, the estimation of tuning width with fMRI might differ due to several methodological factors. First, fMRI has a much poorer spatial resolution than electrophysiology, and each voxel 3.3 mm 3 of cortex contains several thousands of neurons. A voxel containing neurons with many diverse best frequencies would be assigned with a broader width than a voxel containing neurons with more similar best frequencies, which could be reflected in our results. Also, a voxel response may not represent well the heterogeneous responses of many neurons with differently shaped receptive fields, thus introducing noise and imperfection in tuning width estimation. Second, neuronal tuning width may depend on the loudness of the stimuli used (that is there may be nonmonotonic responses to different sound levels). Although most electrophysiological studies have measured tuning width at 10 dB or best level, here we have used much louder (~60 dB) complex sounds. As the tuning of a majority of neurons becomes broader with increasing sound level, a direct comparison across studies is not possible. Third, our tuning width computation reflects the width of the main spectral peak only. As additional spectral peaks in the voxels’ profiles are disregarded by our fitting procedure, voxels with complex profiles would be labelled as narrowly tuned by our method (as long as their main frequency peak is narrow). Consequently, in our measure the tuning width of a region is unrelated to its spectral complexity. In our study, the acquisition of functional data at ultra-high fields (7T) and the experimental design with multiple types of stimuli were key factors for imaging the fine-grained functional organization of a small subcortical structure. FMRI at 7T allowed a significant increase of imaging resolution compared with conventional measurements (3.3 mm 3 compared with the standard 8–27 mm 3 ) and minimizing partial volume effects and contamination between locations with different frequency responses. Although a 1.5 mm isotropic resolution acquisition may be possible also at lower magnetic fields (3T) [16] , the use of high fields presents several advantages. The (supra-linear) increase of the blood oxygen level-dependent effect with field strength resulted in better temporal signal to noise ratio [44] , [45] , and the smaller point spread function at higher fields resulted in more spatially specific responses [46] , [47] . Our study reports functional maps of hIC obtained with both synthetic sounds (‘tones’) and natural sounds. The analysis and interpretation of tonotopic (best frequency) maps obtained using tones are simpler. However, spectrotemporal receptive fields estimated with synthetic sounds have been shown to poorly predict responses to natural stimuli [19] , [48] . We thus considered it important to assess the basic functional properties of the hIC also using natural sounds, which represent a more ecologically valid condition. Importantly, with natural sounds we capitalized on the possibility of resolving the spectral properties of fMRI voxels in a large (and densely sampled) frequency range. Obtaining similar SRPs with synthetic tones would have required excessively long acquisition times (about five times longer sessions than the ones performed here). The increased spectral resolution of the voxels’ SRPs also enabled mapping tuning width in the hIC. Albeit not identical, tonotopic maps obtained from natural sounds were significantly spatially correlated with those obtained with tones, which suggests an overall consistency. Existing differences between the maps may reflect genuine differences in neuronal responses [19] . Alternatively, they may result from the effects of un-modeled acoustic features (for example spectral-temporal modulations) on the estimation of the voxels’ SRPs. Our findings have significant implications for the study of human auditory processing. They enable a comparison of human and animal auditory systems at the subcortical processing level and pave the way to the mapping of relevant acoustic features in the human auditory subcortical pathway. Furthermore, they provide an essential first step for studying the interaction between midbrain and cortex at the fine-grained level of frequency-selective channels. Data acquisition and experimental design The imaging protocol used in this study was approved by the Institutional Review Board (IRB) of the University of Minnesota. Data were acquired on a 7T whole body system driven by a Siemens console using a high-performing head gradient. We acquired anatomical ( T 1 weighted and proton density weighted; 1 mm 3 ) and functional ( T 2 * weighted blood oxygen level-dependent; 1.5 mm 3 ) images in five subjects in Experiments 1 and 2 (three males, two females; two scanning sessions per subject; Supplementary Information ) and four subjects in Experiment 3 (three males and one female). In Experiments 1 and 2, sounds were presented with an MR-compatible audio system based on air tubes (Avotec Inc.) with a linear frequency transfer function up to about 4 kHz. The system was modified in such a way that the final piece of the air tubes was directly inserted in the subjects’ ear through mouldable earplugs. In Experiment 3, sounds were presented with an MR compatible piezoelectric/earbud system (Sensimetric Inc.) with a linear frequency transfer function up to about 8 kHz. In all experiments, sounds were presented at ~60 dB. fMRI data analysis of tonotopic maps Functional and anatomical data were analysed on BrainVoyager QX (see Supplementary Information for details). After preprocessing, a standard general linear model analysis was used to extract responses to the tones in Experiments 1 and 3 (three frequencies and eight frequencies, respectively). Tonotopic maps were obtained by computing ‘best frequency’ maps [13] where colours indicate the frequency eliciting the strongest fMRI response. Tonotopic mapping was limited to the voxels showing a significant response to all sounds (F-test; q[FDR]<0.001; corresponding to p ). For Experiment 2, tonotopic maps were obtained using an fMRI ‘encoding’ method [20] , [21] , [22] , [23] to extract voxels’ SRP in the (0–8 kHz) frequency range binned in forty distinct intervals [31] . Tonotopy maps were obtained from the SRPs colour-coding the frequency interval corresponding to the SRP peak. Statistical significance of the maps was computed using permutation testing (see Supplementary Information for details). The consistency of tonotopic maps obtained with synthetic tones and natural sounds (Experiments 1 and 2) was evaluated using Pearson Correlation (see Supplementary Information for details). To quantify the direction of the main tonotopic gradient, we performed a gradient analysis on the single subject and group hIC tonotopic maps from all experiments separately. Specifically, for each voxel in subsequent sagittal slices we computed the two-dimensional gradient (from low-to-high frequency) of the tonotopic map. The gradient direction, with respect to a transversal (that is horizontal) vector pointing in the anterior-to-posterior direction, was obtained as the angle of the spatial derivative vector at each voxel. To avoid nuisance effect from voxels at the border of the map the direction was averaged within a region of interest obtained eliminating the outer-most shell of the hIC. fMRI data analysis of tuning width maps Tuning width maps were extracted from Experiment 2, as the FWHM of the voxels’ SRP around the maximum response. Statistical significance of tuning width maps was assigned using permutation testing. We computed the percentage of voxels with a specific haemodynamic spectral tuning value in the hIC and in three cortical areas (see Supplementary Information for details). Next, we compared across subjects (1) the mean percentage of voxels within four haemodynamic spectral tuning windows and (2) the mean tuning width using non-parametric statistics (Wilcoxon rank sum test). How to cite this article: De Martino, F. et al. Spatial organization of frequency preference and selectivity in the human inferior colliculus. Nat. Commun. 4:1386 doi: 10.1038/ncomms2379 (2013).